Linear magnetoresistance due to multiple-electron scattering by low-mobility islands in an inhomogeneous conductor Linear transverse magnetoresistance is commonly observed in many material systems including semimetals, narrow band-gap semiconductors, multi-layer graphene and topological insulators. It can originate in an inhomogeneous conductor from distortions in the current paths induced by macroscopic spatial fluctuations in the carrier mobility and it has been explained using a phenomenological semiclassical random resistor network model. However, the link between the linear magnetoresistance and the microscopic nature of the electron dynamics remains unknown. Here we demonstrate how the linear magnetoresistance arises from the stochastic behaviour of the electronic cycloidal trajectories around low-mobility islands in high-mobility inhomogeneous conductors and that this process is only weakly affected by the applied electric field strength. Also, we establish a quantitative link between the island morphology and the strength of linear magnetoresistance of relevance for future applications. Linear transverse magnetoresistance (MR) is a phenomenon commonly observed in many material systems, including semimetals [1] , narrow band-gap semiconductors [2] , [3] , multi-layer graphene [4] and topological insulators [5] . Linear MR can arise from either quantum [6] or classical effects [7] , [8] . In particular, it can originate in an inhomogeneous conductor from distortions in the current paths induced by macroscopic spatial fluctuations in the carrier mobility; this type of non-saturating linear MR has been observed in several materials and explained in terms of a phenomenological semiclassical random resistor network model [7] , [8] . However, the link between the linear MR and the microscopic nature of the electron dynamics remains still unexplored. Existing theories of classical linear MR apply to systems with ohmic conductivity, whereas the effects of hot electron dynamics on the linear MR are largely unknown. On the other hand, a significant enhancement of MR has been observed in the non-omhic space-charge limited transport regime [9] and under avalanche breakdown [10] , thus raising problems of fundamental interest and technological relevance, that is, what is the specific carrier dynamics giving rise to the linear MR, is it preserved in the presence of a large applied electric field and can it be controlled and exploited in sensitive Hall sensors or magnetoresistors [11] ? Here, we examine the physical origin of the classical linear MR in a high-mobility inhomogeneous conductor. Our measurements and Monte Carlo simulations focus on the n -type compound semiconductor InAs and consider an extended range of applied electric ( E ) and magnetic ( B ) fields, and different sample geometries. By modelling our data with Monte Carlo simulations of the electron dynamics, we demonstrate that the linear MR arises from multiple scattering of the current-carrying electrons by low-mobility islands within the conducting layer. This process is only weakly affected by the details of the electronic band structure and electric field strength. Also, it persists at magnetic fields as high as ~50 T corresponding to a magnetic length as small as 4 nm, significantly smaller than the electron mean free path (~100 nm) and island size. The link between the linear MR and the stochastic behaviour of the electronic cycloidal trajectories around low-mobility islands is a finding of general interest as it is relevant to all high-mobility inhomogeneous conductors. The identification of a quantitative link between the island morphology and the strength of linear MR is also potentially useful for tailoring the linear MR in future applications. Material systems and devices Our InAs and In(AsN) epilayers were grown by molecular beam epitaxy (MBE) on a semi-insulating (100)-oriented GaAs substrate. Owing to the mismatch between the substrate and epilayer lattices, inhomogeneities can arise due to the presence of dislocations and defects; also, the N-atoms act as scattering centres for the conduction electrons [12] , [13] . Thus with increasing N-content from 0 to 1%, the electron Hall mobility decreases from μ H =3.3 m 2 V −1 s −1 (3.1 m 2 V −1 s −1 ) to 0.6 m 2 V −1 s −1 (0.5 m 2 V −1 s −1 ) at T =300 K (4.2 K). Correspondingly, the electron density increases from n e =4×10 16 cm −3 in InAs to n e =1.4×10 17 cm −3 in In(AsN), with both values being very weakly affected by temperature. The presence of inhomogeneous disorder combined with the high electron mobility makes these InAs and In(AsN) layers particularly well suited to the study of classical linear MR: even in the low-mobility layers the high values of μB ≫ 1, which are necessary for observing a large MR, can be achieved with available conventional (superconducting) solenoids. To investigate the influence of sample geometry and electric field on the MR, two-terminal planar devices with InAs channels of length L =2, 5 and 10 μm and of width W =1, 2 and 5 μm were also studied. High magnetic field studies In our experiments, the magnetic field was applied parallel to the growth axis z , that is, B =[0, 0, B z ]. The transverse MR ratio defined as Δρ xx / ρ xx =[ ρ xx ( B z )− ρ xx (0)]/ ρ xx (0) was studied with magnetic fields, B z , up to 14 T, generated by a superconducting magnet, or in a pulsed solenoid at B z up to 47 T with a total pulse length of 100 ms. 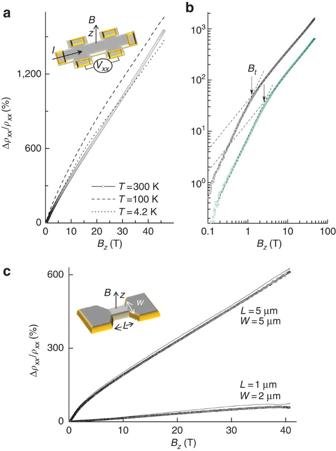Figure 1: Linear transverse MR in Hall bars and short-channel devices. (a) Transverse MR, Δρxx/ρxx, as a function of magnetic field,Bz, for an InAs Hall-bar atT=4.2, 100 and 300 K. (b) Δρxx/ρxxas a function ofBzfor InAs (black) and In(AsN) (green) Hall-bars (T=300 K). Dashed lines and arrows illustrate the transition of the dependence of Δρxx/ρxxonBzfrom quadratic to linear at the characteristic magnetic fieldBzt. A linear fit to the MR data by the relation Δρxx/ρxx=μ0Bz(s/2l) gives an average island coverage factorf~0.17 and 0.32 in InAs and In(AsN), respectively. Here,sis the average size of the low-mobility regions,lis the inter-island separation andμ0is the zero field mobility. (c) Δρxx/ρxxversusBzfor short InAs channels of length,L, and width,W, atT=100 K (line) and 300 K (symbols). The insets in panels (a) and (c) sketch a Hall-bar and a two-terminal planar device, respectively. Figure 1a shows the B z -dependence of Δρ xx / ρ xx for an Hall-bar based on n -type InAs. A positive linear MR is observed at B z >1 T and is weakly affected by temperature in the range T =4.2–300 K. A weak oscillatory component of ρ xx is observed at low temperature ( T <20 K), which we attribute to the Shubnikov–de Haas effect in the two-dimensional electron gas that accumulates on the surface of InAs due to the bending of the conduction band by charged native surface defects [12] . The resistance of the surface two-dimensional electron gas at B z =0 T is at least one order of magnitude higher than ρ xx and, at all values of B z and T , the amplitude of the magneto-oscillations is much smaller than the measured monotonically increasing MR. Figure 1: Linear transverse MR in Hall bars and short-channel devices. ( a ) Transverse MR, Δ ρ xx / ρ xx , as a function of magnetic field, B z , for an InAs Hall-bar at T =4.2, 100 and 300 K. ( b ) Δ ρ xx / ρ xx as a function of B z for InAs (black) and In(AsN) (green) Hall-bars ( T =300 K). Dashed lines and arrows illustrate the transition of the dependence of Δ ρ xx / ρ xx on B z from quadratic to linear at the characteristic magnetic field B z t . A linear fit to the MR data by the relation Δ ρ xx / ρ xx = μ 0 B z ( s/ 2 l ) gives an average island coverage factor f ~0.17 and 0.32 in InAs and In(AsN), respectively. Here, s is the average size of the low-mobility regions, l is the inter-island separation and μ 0 is the zero field mobility. ( c ) Δ ρ xx / ρ xx versus B z for short InAs channels of length, L , and width, W , at T =100 K (line) and 300 K (symbols). The insets in panels ( a ) and ( c ) sketch a Hall-bar and a two-terminal planar device, respectively. Full size image Linear MR can occur when the electron distribution enters the so-called quantum limit, in which only the lowest Landau level is occupied, that is, when the cyclotron energy, , exceeds the Fermi energy, ε F , and when , ε F ≫ k B T [6] (ref. 6 ). As shown in Fig. 1b , the transition of the MR to a linear B -dependence occurs at B z ~1 T below the value satisfying the quantum limit condition , that is, . This limit corresponds to fields >3 T for an electron density n e =4×10 16 cm −3 , which we derive from the gradient of the Hall resistivity, ρ xy , in the limit B z →0. Also, we note that the condition for single occupancy of the lowest Landau level requires that . This condition is satisfied for temperatures <50 K at B z =1 T and for the electron cyclotron mass of InAs ( m e =(0.025±0.01) m 0 , where m 0 is the electron mass in vacuum) [14] . However, the linear MR is observed well above T =50 K (see Fig. 1 ), indicating that it does not have a quantum origin, but is a classical effect. Classical linear MR has been explained using a phenomenological model in which the distorted current paths arising from disorder-induced ihnomogeneities and macroscopic variations, Δ μ , in the electron mobility are simulated by a network of random resistors. Each resistor element has four terminals to take into account not only the local resistive voltage drop but also the Hall voltage associated with the local mobility, μ , of a particular region of the sample [7] , [8] . The crossover of the MR from quadratic to linear B z -dependence is predicted to occur at a characteristic magnetic field , or at B z t = Δμ −1 for Δ μ / > 1, where corresponds to an average of the spatially varying mobility. A comparison of the B z -dependence of Δ ρ xx / ρ xx in our InAs and In(AsN) Hall-bars at T =300 K (see Fig. 1b ) shows that both the value of 1/ B z t and the slope of the MR follow the systematic decrease of μ from 3.3 m 2 V −1 s −1 in InAs to 0.6 m 2 V −1 s −1 in In(AsN). The characteristic magnetic field B z t provides an estimate of the average mobilities = 1/ B z t ~ 1 m 2 V −1 s −1 and 0.5 m 2 V −1 s −1 in the InAs and In(AsN) samples, respectively, which are comparable with those measured by the Hall effect. Also, the MR tends to follow the temperature dependence of μ : in the InAs sample, an increase of T > 4.2 K and up to T ~100 K leads to an increase of μ H from 3.1 to 3.8 m 2 V −1 s −1 followed by a decrease at T >150 K. This variation is caused by the interplay between impurity and phonon scattering and is accompanied by a similar T -dependence of the MR (see Fig. 1a ). Linear MR is also observed in the two-terminal small channel devices, see Fig. 1c . Monte Carlo simulations As our InAs and In(AsN) epilayers are grown on highly lattice-mismatched GaAs, threading dislocations tend to form at the epilayer/substrate interface. The macroscopic (>0.1 μm) inhomogeneities observed by transmission electron microscopy of our samples [15] are likely to induce variations in the electronic properties. We model the effect of such inhomogenities on the electron dynamics by Monte Carlo simulations [16] . As the magnetic field is applied along the z -direction, the magnetic field affects the components of the electron motion in the x – y plane. In our simulation of the two-dimensional electron trajectories, inhomogeneity is introduced by placing low-mobility islands randomly within the x – y plane ( Fig. 2 ). The random spatial profile of the islands, Δ ( x,y ), is generated from the power spectrum of the autocorrelation function ‹ Δ ( r ) Δ ( r ′)›= Δ 2 exp[−| r − r ′| 2 /Λ 2 ], where Λ is the correlation length, r =( x , y ) and r ′=( x′ , y ′). The low-mobility regions R low are then defined according to the relation . This condition determines the fractional area, f , of the sample with low mobility in which electrons undergo scattering at a rate higher than in the remaining high-mobility part of the sample. In a three-dimensional model, the value of f would result from an average of the f -values from various x–y planes of the three-dimensional conducting channel. In the low-mobility regions, we use a scattering rate r island = r i + r e , where r i =1.5×10 12 s −1 and r e =2.5×10 14 s −1 are the elastic and inelastic phonon scattering rates, respectively; elsewhere, the electron drift is mainly limited by inelastic scattering with r ~ r i . The non-parabolicity of the electron energy dispersion of InAs is modelled as , where m e =0.026 m 0 and α =2.2 eV −1 . This form of the energy dispersion occurs in numerous semiconductors, including the narrow gap InSb for which observations of linear MR have been also reported [2] , [3] . The electron velocity, given by , and the wave vector, k , change with time under the action of the Lorentz force, , where E =[ E x , E y , 0] and B =[0,0, B z ] [17] . The Hall field component, E y , is set so that the y -component of the average electron velocity is zero, that is, , consistent with the current flow for our Hall bars. The main findings of our simulations are not changed if we consider a different geometry in which the Hall field is effectively 'shorted out', that is, E y =0. Thus, our analysis applies not only to Hall-bars but also to short channels and Corbino geometries, in which the Hall electric field is fully 'short-circuited' by the contact electrodes. 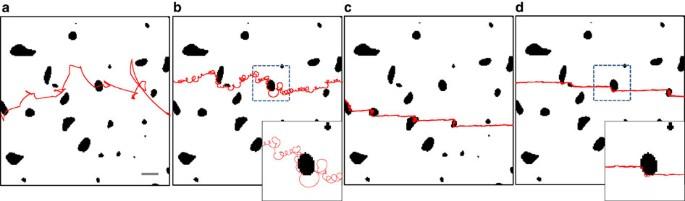Figure 2: Monte Carlo simulations of electron trajectories in magnetic field. Calculated electron trajectories (red lines) in InAs for an applied electric fieldEx=0.5 kV cm−1and under various applied magnetic fieldsBz: (a)Bz=0, (b) 1, (c) 10 and (d) 20 T. The black areas correspond to regions of low mobility. As shown in the magnified trajectories in the insets of panels (b) and (d), in the vicinity of a low-mobility island, the electron undergoes multiple scattering events, which act to deflect the cycloidal motion. The bar in panel (a) corresponds to 1 μm. Figure 2: Monte Carlo simulations of electron trajectories in magnetic field. Calculated electron trajectories (red lines) in InAs for an applied electric field E x =0.5 kV cm −1 and under various applied magnetic fields B z : ( a ) B z =0, ( b ) 1, ( c ) 10 and ( d ) 20 T. The black areas correspond to regions of low mobility. As shown in the magnified trajectories in the insets of panels ( b ) and ( d ), in the vicinity of a low-mobility island, the electron undergoes multiple scattering events, which act to deflect the cycloidal motion. The bar in panel ( a ) corresponds to 1 μm. Full size image Figure 2a–d illustrates the calculated electron trajectories at E x =0.5 kV cm -1 and B z =0, 1, 10 and 20 T. Here, we have assumed a correlation length Λ=0.5 μm, f =5% and low-mobility regions of average size s =0.4 μm and inter-island separation l =8 μm. It can be seen that in the vicinity of the low-mobility islands, the electron undergoes multiple scattering events, which act to deflect the cycloidal motion (see inset of Fig. 2b ). This island-induced scattering is observed at low ( Fig. 2b ) and high ( Fig. 2d ) applied magnetic fields. It is absent in a homogenous system and is responsible for the linear magnetic field dependence of the inverse mobility component, μ xx −1 , whose strength increases with f , as shown in Fig. 3a . 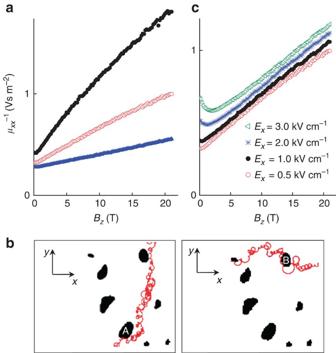Figure 3: Monte Carlo simulations of the electron mobility and its magnetic field dependence. (a) Dependence of the inverse of the mobility,μxx−1on magnetic field,Bz, in InAs at various values of the island coverage factorf=0.1 (black),f=0.05 (red) andf=0.02 (blue). (b) Calculated electron trajectories (red lines) in InAs atBz=1 T,Ex=0.5 kV cm−1and different electric field componentsEy(left:Ey=0 andvy=5×104m s−1; right:Ey=1.5 kV cm−1andvy=0). The black areas show regions of low mobility. A and B indicate two typical islands. (c) Dependence ofμxx−1onExforf=0.05. Figure 3: Monte Carlo simulations of the electron mobility and its magnetic field dependence. ( a ) Dependence of the inverse of the mobility, μ xx −1 on magnetic field, B z , in InAs at various values of the island coverage factor f =0.1 (black), f =0.05 (red) and f =0.02 (blue). ( b ) Calculated electron trajectories (red lines) in InAs at B z =1 T, E x =0.5 kV cm −1 and different electric field components E y (left: E y =0 and v y =5×10 4 m s −1 ; right: E y =1.5 kV cm −1 and v y =0). The black areas show regions of low mobility. A and B indicate two typical islands. ( c ) Dependence of μ xx −1 on E x for f =0.05. Full size image We interpret the results of the Monte Carlo simulations by considering a simplified Drude model of the average electron velocity v x and average hopping distance travelled by the conduction electrons along the x -direction. In a uniform system, that is, with no islands, and for E y =0 and v y ≠0, the average velocity along x is v x= Δ X/τ , where Δ X m e | E x |/( eB z 2 ) is the typical hopping distance and τ is the scattering time. In the presence of inhomogeneity, an electron travels an additional distance Δ X′ ~ s/ 2 around a low-mobility island. As the electron hits an island every time interval τ island ~ l / v H , where v H = E x /B z is the electron Hall velocity along y and l is the distance between the islands, the average electron velocity v x and mobility component μ xx increase as v x =Δ X/τ+ Δ X′/τ island and μ xx =m e /( τe 2 B z 2 ) +s/ (2 lB z ), respectively. Thus, if we compare this result with the case of an homogenous system for which μ xx =m e /( τe 2 B z 2 ) and v x =m e | E x |/( τeB z 2 ), we conclude that at high B z island scattering tends to facilitate electron drift along the x -direction, perpendicular to the cycloidal motion along y (see electron scattering around island A in Fig. 3b ). For the geometry in which E y =0 and v y ≠0, the resistivity component ρ xx is given by . Using the dependence of μ xx on B z at large fields, that is, μ xx ~Δ X′/τ island = s/ (2 lB z ), we derive a linear MR, that is, Δρ xx / ρ xx ~ B z μ *, where μ *= μ 0 ( s/ 2 l ) is and effective mobility and μ 0 is the zero field mobility. A similar conclusion can be drawn for the Hall geometry, that is, for E y ≠0 and v y =0. In this case the resistivity component ρ xx is given by , where μ xy = B z −1 . Using this expression in the limits of high B z , we obtain also in this case that Δ ρ xx / ρ xx ~ B z μ *. Note, however, that in this geometry, the island scattering acts to decrease the average electron velocity, v x , by deflecting the electron motion along y (see electron scattering around island-B in Fig. 3b ). In summary, the magnetic field dependence of the mobility component μ xx due to island scattering generates a characteristic linear dependence of the MR on magnetic field, which is the same in both geometries, that is, E y ≠0 and E y =0. This analysis identifies the physical origin of the random variation of the resistive and Hall effect components of each four-terminal resistive element of the network model [7] , [8] : the randomness arises from the stochastic behaviour of the electronic cycloidal trajectories around the low-mobility islands. From a linear fit to the measured MR data for the large InAs Hall-bar of Fig. 1b by the relation Δρ xx / ρ xx = B z μ *, we obtain μ *=0.33 m 2 V −1 s −1 . For μ 0 = μ H =3.3 m 2 V −1 s −1 , this corresponds to s/ (2 l ) =μ */ μ 0 =0.1 and an average island coverage factor f = s /( s + l )~0.17. Similarly, for the In(AsN) Hall-bar of Fig. 1b we find that s/ (2 l ) =μ */ μ 0 =0.23 and f = s /( s + l )~0.32. Thus, in both cases the average island separation, l, is significantly larger than the average island size, s . Although we cannot deduce the exact value of l or s , we can infer a reasonable estimate from our MR experiments in small channel devices, see Fig. 1c . Here, it can be seen that devices with small values of the channel length L (2–10 μm) and/or width W (1–5 μm) exhibit much smaller values of Δρ xx / ρ xx and in the smallest devices the MR tends to saturate at high B z . The linear MR decreases systematically as the channel width W and length L decrease to values of the order of 1 μm. Thus, we infer that the dimensions of these small devices are comparable to the average island separation. The Monte Carlo simulations indicate that different values of the band non-parabolicity parameter α produce similar linear MR behaviour. Thus, the specific details of the electronic band structure do not have a critical role in the observation of linear MR. Perhaps surprisingly, although μ xx −1 tends to increase with increasing E x , its linear dependence on B z is found to be weakly affected by electric field ( Fig. 3c ) and only at low-magnetic fields (<1 T) and high E x does the value of μ xx −1 tend to decrease with decreasing B z , thus leading to a weak negative MR. This is caused by the interplay between electron cyclotron motion and island-induced scattering, which tends to be increased by E x , that is, electrons hit a low-mobility islands more frequently at higher speeds. However, overall this effect tends to be weak and, at large B z , the deflection of the cycloidal motion by the low-mobility islands and corresponding linear MR are preserved. The weak dependence of the linear MR on applied electric field is confirmed by our MR experiments in the short channel InAs samples. 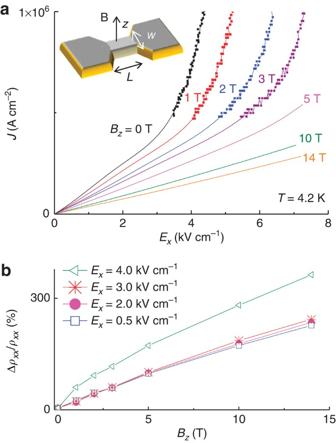Figure 4: Linear transverse MR at high electric fields. (a) Dependence of the current densityJon electric fieldExat various magnetic fieldsBzfor an InAs channel of lengthL=10 μm and widthW=2 μm (T=4.2 K). Measurements of theJ(Ex) characteristics were performed in both the direct current (lines) and pulsed mode (symbols). The inset sketches a two-terminal planar device. (b) Transverse MR,Δρxx/ρxx, as a function ofBzat various values ofEx. The resistivityρxxis calculated asρxx=Ex/J. Figure 4a shows the dependence of the current density J on E x at low temperature ( T =4.2 K) and at various B z (up to 14 T) for an InAs channel of length L =10 μm and width W =2 μm. Similar dependences of J on E x and B z were found in devices with different values of L and W . At B z =0 T, the J ( E x ) curve is approximately linear at low bias. The ohmic behaviour is then followed by a slight sublinear bias dependence and, at larger electric fields, by a sharp rise of the current that is characteristic of systems switching from a state of low to high conductivity due to impact ionization and avalanche breakdown [15] , [18] . At all values of E x , the magnetic field acts to suppress the current and to shift the threshold electric field for impact ionization to significantly higher values. From Fig. 4b , it can be seen that the MR remains linear over an extended range of E x up to ~3 kV cm −1 , just below the threshold electric field for impact ionization. In contrast, in the regime of avalanche breakdown the MR is strongly enhanced and tends to depart from a simple linear dependence due to the effect of the magnetic field in suppressing the avalanche multiplication of carriers [10] . Figure 4: Linear transverse MR at high electric fields. ( a ) Dependence of the current density J on electric field E x at various magnetic fields B z for an InAs channel of length L =10 μm and width W =2 μm ( T =4.2 K). Measurements of the J ( E x ) characteristics were performed in both the direct current (lines) and pulsed mode (symbols). The inset sketches a two-terminal planar device. ( b ) Transverse MR, Δρ xx / ρ xx , as a function of B z at various values of E x . The resistivity ρ xx is calculated as ρ xx = E x /J. Full size image To conclude, our data and analysis indicate that the presence of low-mobility islands in a high-mobility conductor and their effect on the electron trajectories underpin the observation of classical linear MR. We have established a clear link between the stochastic dynamics of the electron trajectory around low-mobility islands caused by multiple scattering at the islands and the classical linear MR in devices with different geometry and size. Although our observations have focused on the high-mobility inhomogeneous n -type InAs and In(AsN) epilayers grown on GaAs, our main findings and conclusions are relevant to a wide variety of structures, device geometries and material systems. Our results are therefore of general interest and will help guiding future research into the manipulation of the linear MR by tuning of the electron trajectories in tailor-made inhomogeneous materials and device structures. Growth and fabrication Our InAs epilayer (thickness t =1. 5 μm) was grown by MBE on a semi-insulating (100)-oriented GaAs substrate. An In(AsN) epilayer ( t =1.3 μm) containing a small concentration (N=1%) of substitutional N-atoms was also grown by MBE using a radio frequency (RF) plasma N-source. The surface reconstruction was monitored by in situ reflection high-energy electron diffraction, while the substrate temperature was measured using an infrared pyrometer calibrated with the surface reconstruction transitions at a fixed As-flux. A Veeco UNI-Bulb RF plasma source was used as nitrogen source. It was set at a RF power of 160 W with a nitrogen flux of 5×10 −6 mbar for all epilayers. The N-content in the In(AsN) epilayers and the crystal quality of the layers were optimized by setting the growth temperature, T G , and the growth rate, r G , to given values in the ranges T G =400–460 °C and r G =0.3–1 μm h −1 , and by keeping a minimum As-flux. The InAs epilayer was grown at T G =460 °C. High-resolution X-ray diffraction measurements using a Bede QC200 diffractometer confirmed a relaxation of the crystal lattice by 98% in the InAs and In(AsN) epilayers. The wafers were spun with photoresist and patterned by photolithography into Hall-bars of length L =1,250 μm and width W =250 μm. Two-terminal planar devices with InAs channels of length L =2, 5 and 10 μm and of width W =1, 2 and 5 μm were also fabricated by electron beam lithography. Each channel was formed by dry-etching the epilayer down to the GaAs substrate. Metal contacts consisting of 10 nm of Ti followed by 200 nm of Au were deposited onto the samples to provide Ti–Au ohmic contacts. Transport studies Measurements of the current–voltage characteristics were performed in both direct current and pulsed mode. For the pulsed mode of acquisition of the current, a voltage pulse generator was used to generate saw-tooth single voltage pulses of duration of 10 μs, and a digital oscilloscope was used for the synchronized and fast temporal recording of the applied bias and current, thus reducing excessive sample heating at high-operating currents. The current–voltage curves in pulsed magnetic field were taken within 1 ms at the top of the magnetic field pulse, during which the magnetic field remains constant to within ±0.5%. How to cite this article: Kozlova, N.V. et al . Linear magnetoresistance due to multiple-electron scattering by low-mobility islands in an inhomogeneous conductor. Nat. Commun. 3:1097 doi: 10.1038/ncomms2106 (2012).